Placental programming of anxiety in adulthood revealed byIgf2-null models Imprinted, maternally silenced insulin-like growth factor-2 is expressed in both the foetus and placenta and has been shown to have roles in foetal and placental development in animal models. Here we compared mice engineered to be null for the placenta-specific P0 transcript (insulin-like growth factor-2-P0 KO) to mice with disruptions of all four insulin-like growth factor-2 transcripts, and therefore null for insulin-like growth factor-2 in both placenta and foetus (insulin-like growth factor-2-total KO). Both models lead to intrauterine growth restriction but dissociate between a situation where there is an imbalance between foetal demand and placental supply of nutrients (the insulin-like growth factor-2-P0 KO) and one where demand and supply is more balanced (the insulin-like growth factor-2-total KO). Increased reactivity to anxiety-provoking stimuli is manifested later in life only in those animals where there is a mismatch between placental supply and foetal demand for nutrients during gestation. Our findings further distinguish placental dysfunction from intrauterine growth restriction and reveal a role for the placenta in long-term programming of emotional behaviour. Prenatal programming of disease risk can occur when exposure to environmental insults in utero lead to enduring changes in function later in life [1] , [2] . Various programming stimuli, such as periods of foetal malnutrition, which result in intrauterine growth restriction (IUGR), are associated with heightened risk for metabolic and cardiovascular disease [3] , [4] , [5] . The long-term consequences of compromised gestation, as indexed by IUGR, also give rise to a range of psychiatric effects [6] , [7] , [8] , including increased risk for emotional disorders [9] , [10] , [11] . The biological mechanisms whereby events occurring before birth can influence emotionality later in life remain unknown. In this work, we examined the role of the placenta in the developmental antecedents of adult behaviour evoked by acute anxiety-inducing circumstances using murine genetic models of disturbed insulin-like growth factor-2 ( Igf2 ) function. Imprinted, maternally silenced Igf2 is expressed in both the foetus and placenta and has been shown to have a major role in foetal and placental development in animal models [12] , [13] . Further, human IUGR has been associated with changes in IGF2 expression in the placenta and foetal circulation of IGF2, although the findings in humans, which are confined to samples obtained at birth, are complex and sometimes contradictory, emphasizing a degree of initial caution in extrapolating between species [14] , [15] , [16] , [17] . In the mouse, there are four main Igf2 transcripts expressed during development: the placental-specific P0 transcript mapping to the labyrinthine trophoblast, the key exchange barrier for nutrients; the P2 and P3 transcripts, expressed in both placenta and foetus; and the P1 transcript expressed mainly in liver [18] . In our experiments we compared mice engineered to be null for the placenta-specific P0 transcript [13] ( Igf2 -P0 KO) with mice with disruptions of all four Igf2 transcripts, and therefore null for Igf2 in both placenta and foetus [19] ( Igf2 -total KO) (see Fig. 1 (ref. 20 )). Previous work has shown that both models lead to IUGR but dissociate between a situation where there is an imbalance between foetal demand and placental supply of nutrients and one where demand and supply is balanced ( Fig. 1 ). In the Igf2 -total KO model, the placental supply of nutrients more equally matches the foetal demand, although both are reduced compared with normal development, whereas in the Igf2 -P0 KO model there is a mismatch between foetal demand and the capability of the placenta to supply nutrition arising from a complex adaptive response, where early increased placental capacity and transport is not sustained and cannot match the foetal demands in late gestation [21] , [22] , [23] , [24] . 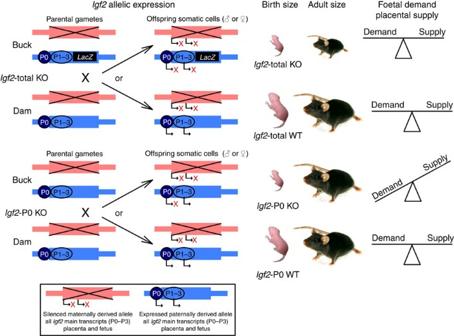Figure 1: Generation ofIgf2-total KO andIgf2-P0 KO mice. Igf2is imprinted with gene expression mainly from the paternal allele of mouse chromosome 7; expression from the maternal allele is attenuated (~5%) excluding the choroid plexus/leptomeninges in brain where expression is bi-allelic57,58.Igf2-total KO mice were created by insertion of aLacZ-targeting vector in the first coding exon abolishing expression of the four mainIgf2transcripts (P0, P1, P2 and P3) in both the placenta and foetus19. This leads to IUGR with the mice remaining small for life19,59. TheIgf2-P0 KO mice were created by deletion of the U2 exon in the P0 promoter region; this prevents production of the placenta-specific P0Igf2transcript but does not interfere with placental or foetal expression of the other mainIgf2transcripts13.Igf2-P0 transcript, which accounts for ~10% of all of placentalIgf2transcripts in late gestation, is the dominant factor during the early stages of placental development and maps to the labyrinthine trophoblast, the key exchange barrier for nutrients18,60. Therefore, attenuation in expression of the P0 transcript leads to significant disruption of normal placental function and IUGR13. However,Igf2transcription is unaffected in the foetus, and once free from the constraints of reduced placental function,Igf2-P0 KO mice eventually reach an equivalent size to WT adults. Thus, although bothIgf2-total KO andIgf2-P0 KO mice are born small, the underlying aetiology of the IUGR in each model differs; inIgf2-total KO mice, foetal demand and placental supply are balanced, but reduced, relative to WT, whereas inIgf2-P0 KO mice an adaptive response occurs, whereby the placenta initially increases the supply capacity but is unable to sustain the adaptation, especially in terms of amino acid transfer, leading to reduced supply, relative to demand, in late gestation21,22,23. To generate the experimental animals, carrier male mice of each line were paired with WT female mice, producing either WT or KO offspring in which the mutations were now present on the paternal allele, and therefore expressed in somatic cells (see Methods for further details). Figure 1: Generation of Igf2 -total KO and Igf2 -P0 KO mice. Igf2 is imprinted with gene expression mainly from the paternal allele of mouse chromosome 7; expression from the maternal allele is attenuated (~5%) excluding the choroid plexus/leptomeninges in brain where expression is bi-allelic [57] , [58] . Igf2 -total KO mice were created by insertion of a LacZ -targeting vector in the first coding exon abolishing expression of the four main Igf2 transcripts (P0, P1, P2 and P3) in both the placenta and foetus [19] . This leads to IUGR with the mice remaining small for life [19] , [59] . The Igf2 -P0 KO mice were created by deletion of the U2 exon in the P0 promoter region; this prevents production of the placenta-specific P0 Igf2 transcript but does not interfere with placental or foetal expression of the other main Igf2 transcripts [13] . Igf2 -P0 transcript, which accounts for ~10% of all of placental Igf2 transcripts in late gestation, is the dominant factor during the early stages of placental development and maps to the labyrinthine trophoblast, the key exchange barrier for nutrients [18] , [60] . Therefore, attenuation in expression of the P0 transcript leads to significant disruption of normal placental function and IUGR [13] . However, Igf2 transcription is unaffected in the foetus, and once free from the constraints of reduced placental function, Igf2 -P0 KO mice eventually reach an equivalent size to WT adults. Thus, although both Igf2 -total KO and Igf2 -P0 KO mice are born small, the underlying aetiology of the IUGR in each model differs; in Igf2 -total KO mice, foetal demand and placental supply are balanced, but reduced, relative to WT, whereas in Igf2 -P0 KO mice an adaptive response occurs, whereby the placenta initially increases the supply capacity but is unable to sustain the adaptation, especially in terms of amino acid transfer, leading to reduced supply, relative to demand, in late gestation [21] , [22] , [23] . To generate the experimental animals, carrier male mice of each line were paired with WT female mice, producing either WT or KO offspring in which the mutations were now present on the paternal allele, and therefore expressed in somatic cells (see Methods for further details). Full size image When we examined adult behaviour in the two models, we found that only IUGR subjects experiencing mismatched supply and demand during gestation, the Igf2 -P0 KO mice, showed alterations in emotionality, exhibiting highly consistent and widespread increases in behavioural indices of anxiety that were accompanied by specific changes in brain gene expression related to emotional behaviours. No effects were seen in the Igf2 -total KO where prenatal supply and demand were more evenly matched, despite these animals suffering a more severe and enduring reduced growth phenotype and completely lacking Igf2 expression throughout the lifespan. Our findings further distinguish placental dysfunction from IUGR per se , and reveal a novel role for the placenta on long-term programming of emotional behaviour, which we hypothesize is dependent on the ability of the placenta to balance the nutritional demands of the foetus. Birth weight and postnatal growth in the Igf2 -KO mice We first established the effects of the Igf2 manipulations on birth weight and postnatal growth. Confirming and extending the original findings of Constância et al . [13] , [19] , in the Igf2 -total KO model, lack of all main Igf2 transcripts in both placenta and foetus led to reduced birth weight, ~55% of wild-type (WT) littermate controls and a reduced physical weight that continued throughout life ( Fig. 2 ). In contrast, the selective absence of placental Igf2- P0 expression in the Igf2 -P0 KO animals, which has been shown to reduce placental nutrient transport mainly during the final trimester of gestation [13] , led to a more moderate IUGR, ~25% of WT littermate control weight and a period of compensatory growth, largely occurring between 25 and 50 days postnatal; these animals attaining near normal size by approximately 100 days old ( Fig. 2 ). 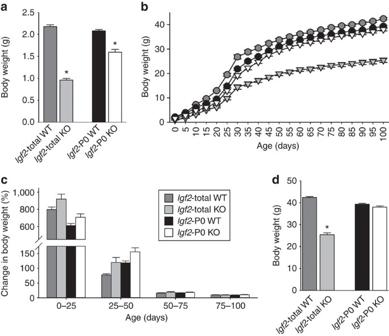Figure 2: BothIgf2-total KO andIgf2-P0 KO mice are born small, butIgf2-P0 KO catch up with WT controls. Mice were weighed every 2 days from birth up to weaning and every 5 days thereafter as an index of growth. Mice of bothIgf2-KO lines had significantly lower birth weights than their WT littermate controls (a, GENOTYPE, F2,135=147.76,P<0.001).Igf2-total KO mice (N=20) exhibited a ~55% reduction in birth weight relative to WT controls (N=39) (post-hoc: F1,96=265.40,P<0.001);Igf2-P0 KO mice (N=40) exhibited a ~25% reduction in birth weight relative to WT controls (N=39) (post-hoc: F1,116=91.78,P<0.001); the comparison betweenIgf2-KO P0 andIgf2-total KO was also significant (post-hoc: F1,58=65.72,P<0.001). Growth curves during the first 100 days of postnatal life are shown inb. (c) Dividing the first 100 days of growth into four equal phases for more detailed analysis of growth rates, theIgf2-total KO mice displayed a significant growth spurt during the first 25 days of postnatal life (GENOTYPE, F2,135=6.65,P<0.001;post-hoc, F1,96=13.19,P<0.001), following which growth rate was not different; however, these mice remained ~38% below WT weight at 100 days old (GENOTYPE, F2,135=182.63,P<0.001;post-hoc, F1,96=365.07,P<0.001) (d).Igf2-P0 KO mice underwent a slightly later main period of accelerated weight gain relative to WT controls (c), between postnatal days 25 and 50 (GENOTYPE, F2,135=10.07,P<0.001;post-hoc, F1,116=19.74,P<0.001). At 100 days old (d), the body weight ofIgf2-P0 KO mice was still significantly reduced in comparison with WT controls (post-hoc, F1,116=21.08,P<0.001); however, this difference reflected only a ~7% reduction compared with the ~25% difference at birth, suggesting a significant period of accelerated compensatory growth. The differences in body weights were maintained throughout the lifespan, as data from older mice (~400 days old) showed a similar pattern (data not shown). Data are for male mice generated from 19Igf2-P0 KO and 18Igf2-total KO litters; ANCOVA was used to analyses all data, co-varying for variance due to the different WT litter-mate control groups. Data are mean+s.e.m., *significant difference from control (α<0.05). Figure 2: Both Igf2 -total KO and Igf2 -P0 KO mice are born small, but Igf2 -P0 KO catch up with WT controls. Mice were weighed every 2 days from birth up to weaning and every 5 days thereafter as an index of growth. Mice of both Igf2- KO lines had significantly lower birth weights than their WT littermate controls ( a , GENOTYPE, F 2,135 =147.76, P <0.001). Igf2- total KO mice ( N =20) exhibited a ~55% reduction in birth weight relative to WT controls ( N =39) ( post-hoc : F 1,96 =265.40, P <0.001); Igf2- P0 KO mice ( N =40) exhibited a ~25% reduction in birth weight relative to WT controls ( N =39) ( post-hoc : F 1,116 =91.78, P <0.001); the comparison between Igf2 -KO P0 and Igf2 -total KO was also significant ( post-hoc : F 1,58 =65.72, P <0.001). Growth curves during the first 100 days of postnatal life are shown in b . ( c ) Dividing the first 100 days of growth into four equal phases for more detailed analysis of growth rates, the Igf2 -total KO mice displayed a significant growth spurt during the first 25 days of postnatal life (GENOTYPE, F 2,135 =6.65, P <0.001; post-hoc , F 1,96 =13.19, P <0.001), following which growth rate was not different; however, these mice remained ~38% below WT weight at 100 days old (GENOTYPE, F 2,135 =182.63, P <0.001; post-hoc , F 1,96 =365.07, P <0.001) ( d ). Igf2- P0 KO mice underwent a slightly later main period of accelerated weight gain relative to WT controls ( c ), between postnatal days 25 and 50 (GENOTYPE, F 2,135 =10.07, P <0.001; post-hoc , F 1,116 =19.74, P <0.001). At 100 days old ( d ), the body weight of Igf2 -P0 KO mice was still significantly reduced in comparison with WT controls ( post-hoc , F 1,116 =21.08, P <0.001); however, this difference reflected only a ~7% reduction compared with the ~25% difference at birth, suggesting a significant period of accelerated compensatory growth. The differences in body weights were maintained throughout the lifespan, as data from older mice (~400 days old) showed a similar pattern (data not shown). Data are for male mice generated from 19 Igf2- P0 KO and 18 Igf2 -total KO litters; ANCOVA was used to analyses all data, co-varying for variance due to the different WT litter-mate control groups. Data are mean+s.e.m., *significant difference from control ( α <0.05). Full size image Selective increases in behavioural anxiety in Igf2 -P0 KO mice To assess emotional function in adulthood, 6-month-old animals were examined in a wide range of established tests assaying emotion-related behaviours [25] , [26] , [27] , [28] . In all cases, the Igf2 -P0 KO mice showed behaviours consistent with increased reactivity to acute anxiety-inducing stimuli; they spent less time on the anxiety-provoking open arms of an elevated plus-maze [29] ( Fig. 3a ), were reluctant to initially enter the exposed central area of an open field and exhibited a greater degree of wall-hugging thigmotaxis behaviour [30] ( Fig. 3c ), were slower to enter a novel environment from one that was familiar to them and overall spent less time in the novel environment [31] ( Fig. 4a ). In addition, Igf2 -P0 KO mice were more wary of consuming a novel foodstuff [32] ( Fig. 4c ) and showed a much greater startle response to a stressful acoustic (120 dB) startle stimulus [33] ( Fig. 4d ). In contrast, the more severely growth-restricted Igf2 -total KO animals were not different to litter-mate WT controls in all tests apart from the open field where this group displayed behaviour consistent with reduced anxiety ( Fig. 3c ). 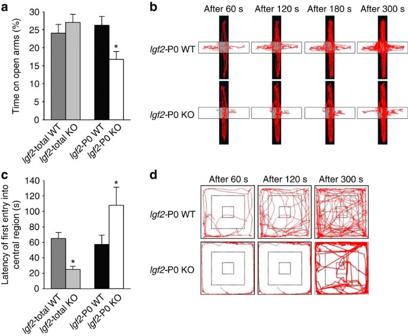Figure 3:Igf2-P0 KO mice show an increase in anxiety in elevated plus-maze and open-field tasks. (a)Igf2-P0 KO (N=21) mice spent less time on the open arms of the elevated plus-maze (EPM), the primary anxiety index in this task, in comparison with WT controls (N=18) andIgf2-total KO mice (N=13) and their WT controls (N=23) (GENOTYPE, F2,72=5.22,P<0.01, effect size eta2=0.14,post-hoc, F1,61=10.07,P<0.01). (b) Video-tracking data illustrating reluctance of a representativeIgf2-P0 KO mouse (bottom) to explore the open arms (shown in white) of the EPM relative to WT (top). (c) Open-field data showingIgf2-P0 KO mice (N=17) were slower to enter the anxiety-provoking, most exposed central area of the apparatus than WT controls (N=18),Igf2-total KO mice (N=11) and WT controls (N=23) (GENOTYPE, F2,62=7.70,P<0.01, eta2=0.16;post-hoc, F1,57=8.90,P<0.02). In contrast,Igf2-total KO mice were quicker to enter this region (post-hoc, F1,31=11.13,P<0.01) (d) Representative activity traces in the open-field demonstrate thatIgf2-P0 KO mice (bottom) showed greater levels of thigmotaxic behaviour (circling round the edge of the open-field) throughout the session and tended to avoid the central anxiety-provoking areas more thanIgf2-P0 WT mice (top). We subjected the data to further statistical analysis, as co-varying for variance in the data due to differences in the litter-mate WT groups was not significant in the initial analysis (ANCOVA,Supplementary Table S3). Using two-way analysis of variance with factors STRAIN (Igf2-P0 orIgf2-total) and GENOTYPE (WT or KO), significant interactions were found for the EPM and open-field data (seeSupplementary Table S4), andpost-hocpairwise analysis showed thatIgf2-P0 KO mice significantly differed from the other three groups of mice (Supplementary Tables S5 and S6). Data are mean+s.e.m., *significant difference from control (α<0.05). Note, data show nominalP-values; theseP-values remained significant, taking into account potential false-discovery rates due to multiple comparisons across all the separate tests of anxiety, as they did for the additional statistical analysis (seeSupplementary Tables S2 and S4). Figure 3: Igf2 -P0 KO mice show an increase in anxiety in elevated plus-maze and open-field tasks. ( a ) Igf2 -P0 KO ( N =21) mice spent less time on the open arms of the elevated plus-maze (EPM), the primary anxiety index in this task, in comparison with WT controls ( N =18) and Igf2 -total KO mice ( N =13) and their WT controls ( N =23) (GENOTYPE, F 2,72 =5.22, P <0.01, effect size eta 2 =0.14, post-hoc , F 1,61 =10.07, P <0.01). ( b ) Video-tracking data illustrating reluctance of a representative Igf2 -P0 KO mouse (bottom) to explore the open arms (shown in white) of the EPM relative to WT (top). ( c ) Open-field data showing Igf2 -P0 KO mice ( N =17) were slower to enter the anxiety-provoking, most exposed central area of the apparatus than WT controls ( N =18), Igf2 -total KO mice ( N =11) and WT controls ( N =23) (GENOTYPE, F 2,62 =7.70, P< 0.01, eta 2 =0.16; post-hoc , F 1,57 =8.90, P< 0.02). In contrast, Igf2 -total KO mice were quicker to enter this region ( post-hoc , F 1,31 =11.13, P< 0.01) ( d ) Representative activity traces in the open-field demonstrate that Igf2 -P0 KO mice (bottom) showed greater levels of thigmotaxic behaviour (circling round the edge of the open-field) throughout the session and tended to avoid the central anxiety-provoking areas more than Igf2 -P0 WT mice (top). We subjected the data to further statistical analysis, as co-varying for variance in the data due to differences in the litter-mate WT groups was not significant in the initial analysis (ANCOVA, Supplementary Table S3 ). Using two-way analysis of variance with factors STRAIN ( Igf2 -P0 or Igf2 -total) and GENOTYPE (WT or KO), significant interactions were found for the EPM and open-field data (see Supplementary Table S4 ), and post-hoc pairwise analysis showed that Igf2 -P0 KO mice significantly differed from the other three groups of mice ( Supplementary Tables S5 and S6 ). Data are mean+s.e.m., *significant difference from control ( α <0.05). Note, data show nominal P -values; these P -values remained significant, taking into account potential false-discovery rates due to multiple comparisons across all the separate tests of anxiety, as they did for the additional statistical analysis (see Supplementary Tables S2 and S4 ). 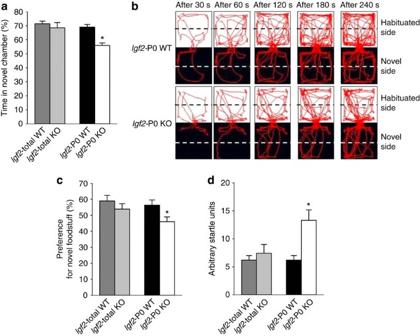Figure 4:Igf2-P0 KO mice show increased anxiety in place preference and food neophobia tasks and increased responses to startling acoustic stimuli. (a) In the novelty place preference (NPP) test,Igf2-P0 KO mice (N=19) spent less time in the unfamiliar and more aversive novel chamber than WT controls (N=22),Igf2-total KO mice (N=9) and WT controls (N=18) (GENOTYPE, F2,64=12.15,P<0.001, eta2=0.16;post-hoc, F1,57=7.55,P<0.05). Although all mice were more wary of entering the novel chamber if it was white in colour (rather than black), the overall statistical pattern remained consistent regardless of chamber colour. (b) Representative video-tracking data illustrating the hesitancy of theIgf2-P0 KO mice (bottom) to enter the novel chamber (grey: habituated/familiar side, black: novel chamber) compared withIgf2-P0 WT mice (top). (c) Further evidence for selective increases in acute anxiety in theIgf2-P0 KO mice (N=36) indexed by increased food neophobia (that is, decreased preference for a novel foodstuff) (GENOTYPE, F2,125=6.59,P<0.03, eta2=0.07;post-hoc, F1,101=4.67,P<0.01), WT controls (N=37),Igf2-total KO mice (N=20) and WT controls (N=30). (d)Igf2-P0 KO mice (N=21) also showed selective enhanced reactivity to stressful acoustic startling stimuli (GENOTYPE, F2,80=7.53,P<0.01, eta2=0.2;post-hoc, F1,67=17.08,P<0.001). WT controls (N=37),Igf2-total KO mice (N=15) and WT controls (N=11). The data were subjected to further statistical analysis, as co-varying for variance in the data due to differences in the litter-mate WT groups was not significant in the initial analysis (ANCOVA,Supplementary Table S3). Using two-way analysis of variance with factors STRAIN (Igf2-P0,Igf2-total) and GENOTYPE (WT, KO), significant interactions were found for the NPP and startle data, but not preference for a novel foodstuff (c), although there was a strong tendency for a significant interaction (seeSupplementary Table S4). Subsequentpost-hocpairwise analysis showed thatIgf2-P0 KO mice significantly differed from the other three groups of mice (Supplementary Table S7–S10). Data are mean+s.e.m., *significant difference from control (α<0.05). Note, data show nominalP-values; theseP-values remained significant, taking into account potential false-discovery rates due to multiple comparisons across all the separate tests of anxiety, as they did for the additional statistical analysis (seeSupplementary Tables S2 and S4). Full size image Figure 4: Igf2 -P0 KO mice show increased anxiety in place preference and food neophobia tasks and increased responses to startling acoustic stimuli. ( a ) In the novelty place preference (NPP) test, Igf2 -P0 KO mice ( N =19) spent less time in the unfamiliar and more aversive novel chamber than WT controls ( N =22), Igf2 -total KO mice ( N =9) and WT controls ( N =18) (GENOTYPE, F 2,64 =12.15, P <0.001, eta 2 =0.16; post-hoc , F 1,57 =7.55, P <0.05). Although all mice were more wary of entering the novel chamber if it was white in colour (rather than black), the overall statistical pattern remained consistent regardless of chamber colour. ( b ) Representative video-tracking data illustrating the hesitancy of the Igf2 -P0 KO mice (bottom) to enter the novel chamber (grey: habituated/familiar side, black: novel chamber) compared with Igf2 -P0 WT mice (top). ( c ) Further evidence for selective increases in acute anxiety in the Igf2 -P0 KO mice ( N =36) indexed by increased food neophobia (that is, decreased preference for a novel foodstuff) (GENOTYPE, F 2,125 =6.59, P <0.03, eta 2 =0.07; post-hoc , F 1,101 =4.67, P <0.01), WT controls ( N =37), Igf2 -total KO mice ( N =20) and WT controls ( N =30). ( d ) Igf2 -P0 KO mice ( N =21) also showed selective enhanced reactivity to stressful acoustic startling stimuli (GENOTYPE, F 2,80 =7.53, P <0.01, eta 2 =0.2; post-hoc , F 1,67 =17.08, P <0.001). WT controls ( N =37), Igf2 -total KO mice ( N =15) and WT controls ( N =11). The data were subjected to further statistical analysis, as co-varying for variance in the data due to differences in the litter-mate WT groups was not significant in the initial analysis (ANCOVA, Supplementary Table S3 ). Using two-way analysis of variance with factors STRAIN ( Igf2 -P0, Igf2 -total) and GENOTYPE (WT, KO), significant interactions were found for the NPP and startle data, but not preference for a novel foodstuff ( c ), although there was a strong tendency for a significant interaction (see Supplementary Table S4 ). Subsequent post-hoc pairwise analysis showed that Igf2 -P0 KO mice significantly differed from the other three groups of mice ( Supplementary Table S7–S10 ). Data are mean+s.e.m., *significant difference from control ( α <0.05). Note, data show nominal P -values; these P -values remained significant, taking into account potential false-discovery rates due to multiple comparisons across all the separate tests of anxiety, as they did for the additional statistical analysis (see Supplementary Tables S2 and S4 ). Full size image The effects on the anxiety phenotypes were highly discrete. The pattern of behaviours in the assays of anxiety could not be accounted for by any underlying differences in general activity levels, motor co-ordination or balance; as evidenced by additional measures taken in the main assays and from a number of separate tests ( Supplementary Figs S1–S5 and Supplementary Table S1 ). Thus, there were no group effects in a range of measures related to activity across the multiple tests; including overall arm entries on the elevated plus-maze ( Supplementary Fig. S1 ), zone entries in the open field ( Supplementary Fig. S2b ) or entries into the novel chamber in the novelty place preference ( Supplementary Fig. S3b ). Furthermore, no group differences were apparent in activity levels monitored separately in activity cages ( Supplementary Fig. S4a ) or in balance and motor co-ordination assessed using the rotarod apparatus ( Supplementary Fig. S4b,c ). Similarly, there were no group differences in the overall amounts of food consumed in the food neophobia assay ( Supplementary Fig. S5b ), indicating the selective neophobic response in the Igf2 -P0 KO mice was not confounded by underlying differences in food consumption per se . Ancillary data from the elevated plus-maze reported in Supplementary Table S1 , specifically, latencies to enter the open-arm, stretch attends and head dips, exploratory behaviours that can also be sensitive to emotional state, did not show any statistically significant group effects, nor did rear in both the elevated plus-maze and open field. Importantly, the anxiogenic effects observed in the Igf2 -P0 KO mice were a mixture of reduced (for example, open-arm exploration in the elevated plus-maze) and increased (for example, startle response) behavioural responding, eliminating the possibility that the behavioural indices of anxiety were confounded by any gross inhibitory or stimulatory effects on behaviour. Moreover, and of major importance to the general experimental design, we were able to take advantage of the paternal expression of imprinted Igf2 to breed male mice carrying a disrupted allele to female WT mice, giving rise to mixed litters of WT and null animals ( Fig. 1 ). This ensured care of normal and manipulated progeny by a common WT mother, in contrast to other models for IUGR that can involve disturbances to both mother and pups [34] , [35] , [36] , thereby minimizing any possibility of early-life maternal effects influencing phenotype and allowing a direct comparison with litter-mate WT controls. Selective effects on brain gene expression in Igf2 -P0 KO mice We then determined whether the behavioural effects were associated with molecular changes in brain using tissue dissected from subjects used in the novelty place preference assay of fear reactivity (for behavioural data, see Fig. 4a ). We focused on the hippocampus (for dissection details, see Supplementary Methods ) and the GABAergic and serotoninergic (5-HT) neurotransmitter systems in light of their established key roles in mediating anxiogenic behaviour [37] , [38] and sensitivity to early-life manipulations [39] , [40] , [41] . Quantitative PCR (see Supplementary Methods ) revealed a highly specific pattern of hippocampal gene expression changes, with significant reductions in expression of the GABAAα3 receptor subunit and 5-HT 2A receptor message in the Igf2 -P0 KO mice ( Fig. 5a ), but not GABAAα2 receptor subunit or 5-HT 1A receptor message ( Fig. 5c ). Both the GABAAα3 receptor subunit and 5-HT 2A receptors are closely linked to the expression of emotional phenotypes [37] , [38] . In line with the anxiety behaviours, the molecular changes in hippocampus were only seen in the Igf2 -P0 KO mice and not in the more severely growth-restricted Igf2 -total KO animals. As an additional element of selectivity, there were no between-group differences in transcript levels in tissue taken from other brain regions, including hypothalamus and striatum ( Fig. 5e ). 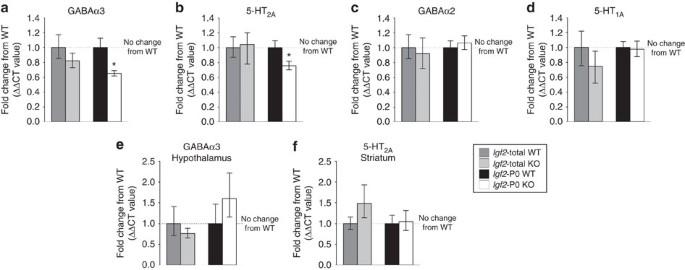Figure 5:Igf2-P0 KO mice show altered expression of genes associated with anxiety in the hippocampus. Hippocampal, hypothalamic and striatal tissue were dissected from the brains of mice that had been behaviourally assessed in the novelty place preference test, and they were subjected to quantitative PCR analysis for the transcript expression of selected gene candidates. Expression levels of the GABAAα3 receptor subunit (t=−2.85,P<0.025, df=14) (a) and the 5-HT2Areceptor (t=−2.33,P<0.05, df=14) (b) genes in the hippocampus were significantly decreased inIgf2-P0 KO mice (N=8) compared withIgf2-P0 WT (N=8), but there were no significant differences in the expression of the GABAAα2 receptor subunit (t=0.02, not significant (n.s.), df=14) (c) or for 5-HT1Areceptor message (t=0.52, n.s., df=14) (d). These effects were regionally specific, as evidenced by equivalent hypothalamic expression of GABAAα3 receptor subunit (t=0.78, n.s., df=14) (e) and striatal expression of 5-HT2Areceptor message (t=0.34, n.s., df=14) (f) betweenIgf2-P0 KO andIgf2-P0 WT. No differences were observed in the expression of any of these genes, in any brain region, betweenIgf2-total WT andIgf2-total KO mice (N=7) and WT (N=11) (hippocampus: GABAAα3t16=1.22, 5-HT2At16=−1.61, GABAAα2t14=0.77 and 5-HT1At16=−0.54; hypothalamus: GABAAα3t15=0.84, striatal 5-HT2At12=−1.51; all n.s). Data are mean±s.e.m., *significant difference from control (α<0.05), allP-values were adjusted with Bonferroni correction for multiple comparison testing. Figure 5: Igf2 -P0 KO mice show altered expression of genes associated with anxiety in the hippocampus. Hippocampal, hypothalamic and striatal tissue were dissected from the brains of mice that had been behaviourally assessed in the novelty place preference test, and they were subjected to quantitative PCR analysis for the transcript expression of selected gene candidates. Expression levels of the GABAAα3 receptor subunit ( t =−2.85, P <0.025, df=14) ( a ) and the 5-HT 2A receptor ( t =−2.33, P <0.05, df=14) ( b ) genes in the hippocampus were significantly decreased in Igf2 -P0 KO mice ( N =8) compared with Igf2 -P0 WT ( N =8), but there were no significant differences in the expression of the GABAAα2 receptor subunit ( t =0.02, not significant (n.s. ), df=14) ( c ) or for 5-HT 1A receptor message ( t =0.52, n.s., df=14) ( d ). These effects were regionally specific, as evidenced by equivalent hypothalamic expression of GABAAα3 receptor subunit ( t =0.78, n.s., df=14) ( e ) and striatal expression of 5-HT 2A receptor message ( t =0.34, n.s., df=14) ( f ) between Igf2 -P0 KO and Igf2 -P0 WT. No differences were observed in the expression of any of these genes, in any brain region, between Igf2 -total WT and Igf2 -total KO mice ( N =7) and WT ( N =11) (hippocampus: GABAAα3 t16 =1.22, 5-HT 2A t16 =−1.61, GABAAα2 t14 =0.77 and 5-HT 1A t16 =−0.54; hypothalamus: GABAAα3 t15 =0.84, striatal 5-HT 2A t12 =−1.51; all n.s). Data are mean±s.e.m., *significant difference from control ( α <0.05), all P -values were adjusted with Bonferroni correction for multiple comparison testing. Full size image The data revealed a consistent pattern of enhanced anxiety responses, coupled with changes in molecular indices of emotional behaviour that were confined to the Igf2 -P0 KO mice. Anxiety is not a unitary concept [26] , [27] , and two main distinctions that have been made are between ‘state’ and ‘trait’ anxiety; the former a transient response, the latter a pervasive condition, as in chronic generalized anxiety disorder in humans. Firm conclusions as to the precise nature of the anxiety phenotypes displayed by the Igf2 -P0 animals are problematical because of the difficulties inherent in making comparisons between human and animal constructs of anxiety; however, insofar, as many of the behavioural tests monitored transitory effects, the present data may be of most relevance to acute anxiety states rather than to any long-term stable trait. As both Igf2 -P0 KO and Igf2 -total KO animals were born small because of IUGR, with the Igf2 -total KO animals remaining small throughout life, neither IUGR per se nor simply being small could explain the pattern of findings. Similarly, the findings cannot be due solely to of lack of Igf2 -P0 expression in the labyrinthine trophoblast of the placenta, because this feature was common to both Igf2 -P0 KO and Igf2 -total KO models. Instead, we suggest that the evidence is most consistent with the conclusion that the brain and behavioural phenotypes seen in the adult Igf2 -P0 KO mice were related, primarily, to compromised exchange functions of the placenta in the face of intact Igf2 action in the foetus, leading in turn to an imbalance between foetal demand and placental supply of nutrients during gestation in these animals. As epidemiological studies in people are retrospective in nature, it is difficult to tease apart the varying environmental factors that underlie IUGR, or to dissociate between effects of different environmental factors and IUGR. Work in animal models inducing IUGR by various manipulations of maternal nutrient supply, for example, uterine artery ligation, low protein diets and hypoxia, do allow an enhanced degree of experimental control relative to human studies [35] , [36] . However, all such experimental studies involve manipulations to the pregnant dam followed by subsequent analysis of function in the offspring and are therefore subject to potential effects arising from changes in postnatal maternal behaviour and dam–pup interactions that may confound any in utero effects [34] . In addition, these models are not optimized for determining the specific contribution of changes in placental function to phenotypes observed in the offspring. In the models that we used, we were able to both avoid maternal effects by generating mixed litters of WT and null animals cared for by a common unaffected WT mother and isolate Igf2 effects in placenta by taking advantage of the selective disruption of the placental-specific Igf2 -P0 transcript. An important question is how the long-range effects of an imbalance of foetal demand and placental supply of nutrients could have an impact on anxiety states and brain function later in life. Acute manipulations of Igf2 in adults have been shown to regulate neurogenesis in brain and have an impact on fear-related behaviour [42] , [43] , [44] ; however, these effects are, a priori , difficult to reconcile with the selective pattern of effects seen here, as Igf2 expression is intact in Igf2 -P0 KO adult mice. Other factors such as differences between the models arising from the lack of imprinting of Igf2 in choroid plexus and leptomeninges of the brain can also be discounted, because this would affect the Igf2 -total KO mice (leading to a 50% reduction of Igf2 expression in these tissues), but not the Igf2 -P0 KO mice. It is also difficult to see how effects on the recently discovered role of placentally synthesized 5-HT in mediating foetal brain development [45] would influence Igf2 -P0 KO mice selectively. Placental Igf2 -P0 has several known functions including the regulation of calcium transport [46] and nutritional transfer across the placenta, especially via the system A amino acid transporter [13] , [22] , which is also downregulated in many human and animal IUGR studies [47] . A role for nutrient-sensitive mechanisms in the developing Igf2 -P0 KO brain, such as amino acid uptake systems [48] , might also be considered. However, whether any of these mechanisms represent a plausible substrate for the behavioural and neurobiological changes that we observed, and how they might interact with the fluctuating conditions of nutrient supply during gestation because of lack of placental P0, has yet to be established. Similarly, a degree of caution is required in direct extrapolation of data obtained from mouse models in humans, especially as P0 transcript expression is not completely confined to the placenta in humans [49] . Although placental effects are likely to be the ultimate cause of the emotional phenotypes displayed by the Igf2 -P0 KO mice, it cannot be discounted that more proximate influences, arising secondarily from the prenatal nutritional imbalance, may also have a role later in development, for example, during the more substantial postnatal ‘catch-up’ growth experienced by Igf2 -P0 KO mice, relative to Igf2 -total KO mice. Similarly, developmental effects on brain areas other than hippocampus may have contributed to the observed behavioural differences. Irrespective of the intermediate pathways linking placenta to adult emotionality, our findings highlight the importance of imprinted gene effects on prenatal nutrient imbalance, and the placenta as a dynamic factor in matching foetal demand to maternal supply, on long-term behavioural dispositions. Subjects Production of Igf2- P0 KO and Igf2 -total KO mice, which were backcrossed to a C57BL/6 background, has been described previously [13] , [19] . To generate the experimental animals, carrier male mice of each line (which did not express the Igf2 mutations in somatic cells because of matrilineal inheritance of the mutated allele) were paired with unmanipulated female CD1 mice (Harlan Olac, UK) producing either WT or KO offspring in which the mutations were now present on the paternal allele and therefore expressed in somatic cells. Outbred female CD1 mice were used as they have large litter sizes and are good mothers. It is also worth reiterating that the dams for each litter were not affected directly by any genetic manipulation or experimental intervention during the pre- and post-natal periods. Igf2 -total KO mice were identified based on their body weight as adults (~20–40% lighter than their WT littermates, Fig. 2 ), whereas Igf2 -P0 KO mice were identified using PCR analysis of DNA extracted from a tail biopsy sample made at weaning; genotypes were confirmed by a second analysis at the end of the experiment (see Supplementary Methods ). In total, four cohorts of mice were used in the subsequent studies (for N , see Figure legends): cohort 1 was used in the birth-weight study, elevated plus-maze and open-field experiments, cohort 2 for the novelty place preference test and the gene analysis, cohort 3 for the startle response assessment and the cohort 4 was also used in the birth-weight study and for the assessment of locomotor activity and motor co-ordination assessment on the rotarod. Mice in cohort 1 and 4 were used for the food neophobia test. Mice from the first and fourth rounds of breeding were weighed on alternate days from birth to weaning, and weekly from then on. Male mice were used in the experiments and were kept in littermate groups through the duration of study (2–5 mice per cage, including at least one representative of each genotype, that is, KO and WT mouse). Home cages were environmentally enriched with cardboard tubes and kept in a temperature and humidity-controlled vivarium (21±2 °C and 50±10%, respectively) with a 12-hour light-dark cycle (lights on at 0700 hours/lights off at 1900 hours). Standard rodent laboratory chow and water were available at libitum unless otherwise stated. All procedures were performed in accordance with the requirements of the UK Animals (Scientific Procedures) Act (1986). General behavioural methods Testing took place between 1000 and 1700 hours, with equal distribution of testing for subjects of different genotypes throughout the day. Mice were habituated to the dimly lit test room for 30 min before testing. Each of the test methods used to assess anxiety involved individual testing of mice; hence, apparatus was cleaned thoroughly with a 2% acetic acid solution between subjects. Data for the elevated plus-maze, open-field and novelty place preference were collected using EthoVision Observer software (Noldus Information Technology, The Netherlands) via a video camera mounted above the centre of each piece of apparatus and each piece of apparatus that was divided into specific virtual zone configurations (see Figs 3 and 4 ). Tracking of each subject, determined as the location of the greater body proportion (12 frames per second), was calibrated for each piece of apparatus before testing using mice of the same body size and fur colour as the experimental subjects. Manual analysis of pilot sessions for each experiment confirmed the accuracy of the tracking software, and all traces were examined for tracking-related artifacts before analysis. The elevated plus-maze The maze, positioned 300 mm above the floor and illuminated evenly at 15 lux, was constructed of white Perspex and consisted of two exposed open arms (175 × 78 mm 2 , length × width) and two equally sized enclosed arms, which had 150-mm high walls [50] . Equivalent arms were arranged opposite to one another ( Fig. 3 ). Subjects were placed at the centre of the maze facing one of the open arms and allowed to freely explore for 5 min. Data from each pair of arms were combined to generate single open- and closed-arm values (number of arm entries, time spent and latency of first entry to each arm and the number of rears). In addition, the following parameters were manually scored for a subset of the cohort: number of stretch-attend postures (defined as an animal keeping its hindquarters in the closed arms but stretching forwards onto an open arm) and number of head dips from the open arms (looking over the edge of an open arm). The open-field The apparatus consisted of a square-shaped arena (750 × 750 mm 2 , length × width), constructed of white plastic and illuminated evenly at 15 lux [50] . Subjects were placed facing the centre of one of the walls and allowed to explore the apparatus for 10 min. The open field was subdivided into three virtual concentric squares ( Fig. 3 ), and the proportion of time spent exploring the central region (a 400 * 400 mm area), the frequency of entries and the latency to first entry the inner-square (200 × 200 mm 2 area), the time spent in the periphery (within 350 mm of each wall) and the number of rears were calculated. Novelty place preference The apparatus consisted of two square Perspex chambers (300 × 300 × 300 mm 3 , width × length × height), one white and the other black, connected by a doorway (70 × 70 mm), which could be blocked ( Fig. 4 ). To enhance the tactile discrimination of the two chambers, coarse grained sandpaper was placed on the floor of one chamber before the start of a session [50] . Mice were habituated to just one chamber (pseudo-randomly selected, and counter-balanced between genotypes) for 45 min; subjects were placed in the centre of the habituated chamber facing away from the closed communicating doorway. Before the 8-min test session, the mouse was removed from the apparatus and the apparatus was cleaned with 2% acetic acid solution, and the sandpaper used to line the floor in one of the chambers was replaced. In the test session, the mice could freely explore both the chambers. All mice were more wary of entering the white chamber when it was novel (~63% preference cf . ~70% preference for the black chamber; for all subjects, main effect of SIDE F 1,64 =8.58, P <0.01), but the overall neophobic effect was consistent whichever side was novel; therefore, data for both chambers were collated before analysis. The number of entries, latency of first entry and the proportion of time spent in the novel compartment were calculated. Assessment of food neophobia To increase the motivation to drink, the mice were placed on a schedule of restricted access to home cage water (2 h per day) for 2 weeks. Small chambers (285 × 130 × 12 mm 3 , length × width × height) in which two small containers (maximum volume ~3 ml each) positioned towards the rear of each chamber were used. There was a single 10-min session each day [32] . In the first two sessions, both containers were filled with water, and in the subsequent four sessions the mice were presented with a choice between water and a 10% condensed milk solution (that is, the novel foodstuff), locations of which were alternated between days. The liquid containers were weighed before and after each session, and the difference was calculated; thus, individual and total volumes for water and condensed milk consumption were calculated. Consumption was normalized for body-weight differences using Kleiber’s 0.75 mass exponent [51] , and the preference for condensed milk was calculated as a percentage of total consumption for each of the final 4 days of testing. Assessment of acoustic startle response The startle chamber apparatus consisted of a ventilated and soundproofed SR-LAB startle chamber (San Diego Instruments, CA, USA) containing a non-restrictive Plexiglas cylinder (35 mm in diameter), mounted on a Perspex plinth, into which a single mouse was placed. The motor responses of subjects to white noise stimuli (generated from a speaker 120 mm above the cylinder) were recorded via a piezoelectric accelerometer, attached centrally below the Plexiglas cylinder, which converted flexion plinth vibration into electrical signals [52] . Startle responses were monitored for 65 ms following the onset of the stimulus. A session consisted of a 5-min habituation phase (background noise of 70 dB, [A] scale) followed by exposure to 12,120 dB stimuli (0.3 s duration), presented with a 10 s random interval (range 6 s to 14 s). Acoustic startle response was normalized for body-weight differences using Kleiber’s 0.75 mass exponent [51] . Quantitative PCR methodologies for analysis of gene expression Tissue from a sample of mice for each genotype of the Igf2 -total and Igf2 -P0 lines that were assessed in the novelty place preference assay of fear reactivity was used to assess gene expression using standardized quantitative PCR methods (see Supplementary Methods ), with quantification using the 2 −ΔΔCt method [53] . Based on the pattern of behavioural findings, only selected brain regions were analysed for specific gene candidates (see main text). Samples were run in triplicate, and the final C t values were averaged. The change in expression of the target genes, after normalization to the two house-keeping genes (Δ C t), was transformed to yield 2 −ΔΔ C t values used for subsequent analysis [54] . C t values were derived from a log-linear plot of the PCR signal against the cycle number, which depicts the C t value as an exponential instead of a linear term, hence the transformation [55] , [56] . Relative changes from WT expression were calculated for each target gene and also transformed. Statistical analysis All statistical analyses were carried out using SPSS 18.0 (IBM, USA). Data for each behavioural test were analysed by separate analysis of covariance (ANCOVA) with a main between subject factor of GENOTYPE (WT, Igf2 -P0 KO, Igf2 -total KO) and co-varying for the different line origins of the WT groups (necessary to account for the fact that the Igf2 -P0 KO, Igf2 -total KO mice were generated from separate lines with their own WT littermate controls). Within-subject factors were designated for each test as appropriate, for example, ARM (open/closed arms) for the elevated plus-maze, ZONE (inner/middle/outer zones) of the open field, habituated/novel chambers of the novelty place preference test and SESSION for the novel food consumption. In each analysis, the effect of the covariate was nonsignificant ( Supplementary Table S3 ); therefore, these data were also analysed using a two-way analysis of variance with factors of STRAIN ( Igf2 -P0, Igf2 -total) and GENOTYPE (WT, KO) (see Supplementary Table S4 for details). The significance of the interaction term was used to assess whether the difference between Igf2 -P0 KO group and the WT group was significantly different from the difference between Igf2 -P0 KO and the Igf2 -total KO groups (see Supplementary Tables S5–S10 ). Birth weight and early postnatal growth were analysed using either ANCOVA, with factor of GENOTYPE for cross-sectional genotype differences, or with factors of GENOTYPE and repeated-measure factor of AGE for the main growth curve. Post-hoc pairwise comparisons were performed using the Bonferroni test, with alpha values of <0.05 regarded as significant. Skewed data were transformed by either log 10 ( x +1) or arcsine transformations before ANCOVA, and Greenhouse-Geisser degrees of freedom corrections were applied as necessary to repeated-measures factors in relevant ANCOVAs (nominal values for the relevant degrees of freedom are reported). Behavioural data were subjected to Benjamini and Hochberg False-Discovery Rate analysis for multiple comparisons effects. Gene expression data were analysed using independent-samples t -tests, followed by Bonferroni correction for multiple comparisons. How to cite this article: Mikaelsson, M. A. et al . Placental programming of anxiety in adulthood revealed by Igf2 -null models. Nat. Commun. 4:2311 doi: 10.1038/ncomms3311 (2013).